Ammonia as a case study for the spontaneous ionization of a simple hydrogen-bonded compound Modern ab initio calculations predict ionic and superionic states in highly compressed water and ammonia. The prediction apparently contradicts state-of-the-art experimentally established phase diagrams overwhelmingly dominated by molecular phases. Here we present experimental evidence that the threshold pressure of ~120 GPa induces in molecular ammonia the process of autoionization to yet experimentally unknown ionic compound—ammonium amide. Our supplementary theoretical simulations provide valuable insight into the mechanism of autoionization showing no hydrogen bond symmetrization along the transformation path, a remarkably small energy barrier between competing phases and the impact of structural rearrangement contribution on the overall conversion rate. This discovery is bridging theory and experiment thus opening new possibilities for studying molecular interactions in hydrogen-bonded systems. Experimental knowledge on this novel ionic phase of ammonia also provides strong motivation for reconsideration of the theory of molecular ice layers formation and dynamics in giant gas planets. Typically, molecular compounds in condensed phase exhibit primarily strong covalent intramolecular and secondary weak (that is, van der Waals) intermolecular bonds. External compression to higher densities is expected to promote phase transformations in which electrons within intramolecular bonds delocalize to form extended covalent framework or polymeric solids, at intermediate pressure ranges, and metallic phases at higher pressures [1] , [2] , [3] , [4] , [5] , [6] , [7] . In fact, transformation of a simple molecular compound to an ionic solid upon compression is a very rare phenomenon. So far, the only experimentally confirmed example is the formation of nitrosonium (NO + ) nitrate (NO3 − ), which forms from molecular nitrogen oxides (N 2 O (refs 8 , 9 , 10 ), mixture of NO and NO 2 (ref. 11 ), N 2 O 4 (refs 12 , 13 , 14 , 15 )) or N 2 /O 2 mixture [16] , [17] . In this particular case, depending on the initial substrate, the autoionization process requires higher pressure, elevated temperature and/or specific irradiation of visible, infrared (IR) or X-ray wavelength range. At such conditions, disintegration of molecules is induced promoting the formation of ionic compounds via a radical-mediated mechanism. Ammonia belongs to an important group of archetypal binary compounds forming molecular hydrogen-bonded (HB) solids. On the one hand, state-of-the-art experimentally established phase diagrams of HB solids (H 2 O, NH 3 , H 2 S, HHal (Hal=Cl, Br, I)) prove the exclusive domination of molecular forms. On the other hand, modern theoretical studies intriguingly predict new forms of water and ammonia with partial or complete charge separation. Ionic forms are predicted to be stable at room temperature and pressure as high as ~1,500 GPa and ~90 GPa for water [18] and ammonia [19] , respectively. It has been also predicted that at certain high-pressure/high-temperature (HT/HP) conditions water and ammonia become a protonic conductor in which the hydrogen atoms undergo rapid hops between neighbouring molecules forming a superionic solid or ionic fluid [20] . Two recent attempts aiming at verification of the later prediction in ammonia provided contradicting conclusions making definitive experimental confirmation of new superionic form elusive [21] , [22] . Here we undertake extensive experimental and theoretical studies in the broadest pressure range ever considered before (from ambient to 300 GPa) including X-ray diffraction (XRD), IR absorption and Raman scattering measurements, in order to explore the possible existence of hypothetical thermodynamically stable, but hitherto experimentally not confirmed high-pressure forms of ammonia. On the basis of obtained results, we report experimental proofs of the pressure-induced formation of ammonium amide (NH 4 + NH 2 − ) along with the theoretical elucidation of the autoionization process in molecular ammonia under pressure. Structural study We started our studies from the pressure region for which phase composition and properties of ammonia are relatively well established. At pressure of 70 GPa, our X-ray diffraction studies performed on polycrystalline samples revealed diffraction patterns corresponding to the molecular form of ammonia crystallizing in the P2 1 2 1 2 1 space group. In our XRD study, the stability region of the P2 1 2 1 2 1 form was confirmed in the pressure range up to ~114 GPa, in agreement with previously reported experimental data [23] . Upon further compression a gradual, but pronounced redistribution of measured intensities was observed that along with distinct splitting of one particular reflection indicated substantial structural changes ( Fig. 1a ). The observed diffraction patterns at pressures above 128 GPa could not be assigned to solely P2 1 2 1 2 1 symmetry suggesting the formation of a new phase. Although the measured angular range (2θ) was insufficient to derive an exact structure solution, diffraction patterns above 135 GPa were consistent with the assumed coexistence of two phases: the one of P2 1 2 1 2 1 and the other of Pma2 symmetry ( Fig. 1a,d,e ). Moreover, the pressure evolution of hkl(400) and hkl(011) reflections (the ‘Δ’splitting) was also consistent with theoretically calculated for Pma2 structure ( Fig. 1b,c ). In recent density-functional-theory (DFT) study, the same Pma2 symmetry has been suggested for an ionic phase, thermodynamically stable already above 90 GPa [19] , although it was not experimentally confirmed in the previous study performed on a single crystal up to 123 GPa [23] . 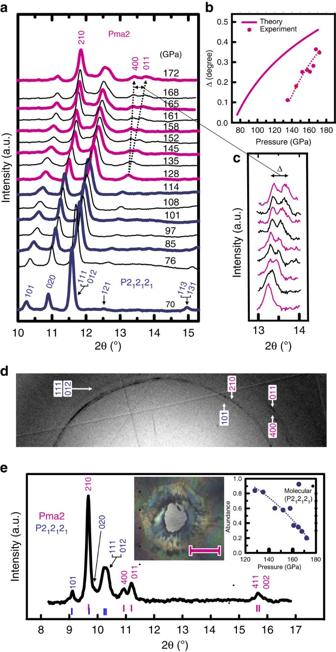Figure 1: Structural study of solid ammonia under pressure. (a) Representative room temperature X-ray diffraction patterns at various pressure acquired at HPCAT beamline (λ=0.4125 Å). Reflections belonging to P212121and Pma2 are marked blue and magenta, respectively. Arrows are an eye guide for evolution of reflections hkl(400) and hkl(011) belonging to Pma2 space group proposed in ref.19. (b) Enlarged view of XRD patterns. Splitting is defined as ‘Δ’ – difference between the position of hhl(011) and hkl(400) reflections. (c). Pressure evolution of splitting. Comparison of calculated and experimentally measured data (dot curve is an eye guide). (d) Fragment of the experimental 2D CCD diffraction image corresponding to the integrated pattern shown ine. (e) Room temperature XRD pattern acquired at GSECARS beamline (λ=0.3,344 Å). Reflections (hkl)=(400) and (011) are clearly resolved. Black curve represents integrated experimental XRD pattern, blue (royal) and magenta curves correspond to calculated patterns for P212121and Pma2 structure, respectively. The same applies to tick marks. Inset (left): a representative microphotograph of a sample chamber filled with solidified transparent ammonia taken under combined transmitted and reflected illumination at pressure 172 GPa. Gasket material was tungsten. Length of the scale bar corresponds to 50 μm. Inset (right): pressure evolution of the abundance of P212121phase (estimation is based on the analysis of experimental and calculated XRD patterns). Figure 1: Structural study of solid ammonia under pressure. ( a ) Representative room temperature X-ray diffraction patterns at various pressure acquired at HPCAT beamline ( λ =0.4125 Å). Reflections belonging to P2 1 2 1 2 1 and Pma2 are marked blue and magenta, respectively. Arrows are an eye guide for evolution of reflections hkl(400) and hkl(011) belonging to Pma2 space group proposed in ref. 19 . ( b ) Enlarged view of XRD patterns. Splitting is defined as ‘Δ’ – difference between the position of hhl(011) and hkl(400) reflections. ( c ). Pressure evolution of splitting. Comparison of calculated and experimentally measured data (dot curve is an eye guide). ( d ) Fragment of the experimental 2D CCD diffraction image corresponding to the integrated pattern shown in e . ( e ) Room temperature XRD pattern acquired at GSECARS beamline ( λ =0.3,344 Å). Reflections (hkl)=(400) and (011) are clearly resolved. Black curve represents integrated experimental XRD pattern, blue (royal) and magenta curves correspond to calculated patterns for P2 1 2 1 2 1 and Pma2 structure, respectively. The same applies to tick marks. Inset (left): a representative microphotograph of a sample chamber filled with solidified transparent ammonia taken under combined transmitted and reflected illumination at pressure 172 GPa. Gasket material was tungsten. Length of the scale bar corresponds to 50 μm. Inset (right): pressure evolution of the abundance of P2 1 2 1 2 1 phase (estimation is based on the analysis of experimental and calculated XRD patterns). Full size image In view of these results, further experimental characterization of spectroscopic properties of the observed new phase was required. For that purpose, we implemented IR absorption and Raman scattering techniques. In addition, following the theoretical suggestion from the ref. 19 , we repeated DFT study for ammonia under pressure. We considered the thermodynamic stability of the known molecular (P2 1 2 1 2 1 ) and the proposed ionic (Pma2) phases as a function of pressure. Having reproduced the previously reported relation between the enthalpies of both phases, we further performed group theory analysis to calculate optical phonon and molecular vibration spectra (both IR and Raman active) and their evolution under pressure. Most remarkable changes in the optical spectra (both IR and Raman) were observed in the 126–133 GPa pressure range correlating with pressures at which major changes in the XRD patterns also took place. Although optical spectra changed substantially in the whole measured spectral range ( Supplementary Fig. 1A–C ), we found it instructive to describe here only the most pronounced changes. IR absorption Despite relatively low resolution of the measured spectra unavoidable for ammonia, the most pronounced new feature was the appearance of a broad and intensive absorption band in the wavenumber range from ~1,800 to ~2,700 cm −1 ( Fig. 2a,b and Supplementary Fig. 2A,B and Supplementary Discussion ). Another major indication of phase transition was observed in the region>3,000 cm −1 —the range of high-frequency molecular vibrons, which initially were associated solely with ‘N–H’ stretching modes of NH 3 molecules (with the maximum centred near 3,500 cm −1 ). Under external pressure, that group clearly shifted to the lower frequency region centred at ~3,250 cm −1 . Having compared the measured and calculated spectra, we associate the new broadband of enhanced absorption (centred at ~2,250 cm −1 ) with the lower frequency group of NH 4 + -derived vibrons. At the same time, the appearance of additional absorption related to ‘N–H’ stretching modes related to NH 4 + and NH 2 − ions ( Fig. 2c ) accounts for the red shift (shift to lower frequencies) of measured signal>3,000 cm −1 that formerly has been associated exclusively with ‘N–H’ stretching of NH 3 molecules. 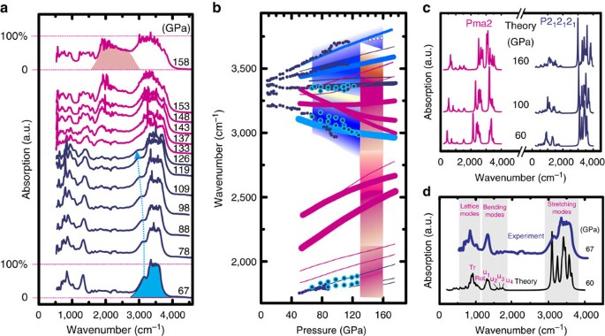Figure 2: IR absorption study of solid ammonia under pressure. (a) Representative room temperature IR absorption spectra at various pressures. Colours depict features attributed to molecular phase (blue (royal)) and ionic (magenta) phases, respectively. The spectral region of ‘N–H’ stretching band corresponding to molecular phase is highlighted blue. New band of strong absorption not related to the molecular phase is highlighted pink. Blue arrow is an eye guide for pressure evolution of the soft ‘N–H’ stretching mode due to hydrogen bonding. (b). Pressure evolution of the measured positions of signals in the wavenumber range from 1,800–4,000 cm−1. Symbols represent experimental data while lines represent calculated data from ref.19. Line thickness corresponds to signal intensity. Solid dark blue symbols correspond to experimental data reported in ref.24while solid light blue outlined symbols represent data measured in this work. Blue and magenta highlighted fields correspond to measured strong absorption associated with the molecular and the ionic phase respectively. (c) Comparison of theoretically calculated IR absorption spectra and their evolution with pressure. (d) Comparison of IR absorption spectra measured at 67 GPa and calculated at 60 GPa. Figure 2: IR absorption study of solid ammonia under pressure. ( a ) Representative room temperature IR absorption spectra at various pressures. Colours depict features attributed to molecular phase (blue (royal)) and ionic (magenta) phases, respectively. The spectral region of ‘N–H’ stretching band corresponding to molecular phase is highlighted blue. New band of strong absorption not related to the molecular phase is highlighted pink. Blue arrow is an eye guide for pressure evolution of the soft ‘N–H’ stretching mode due to hydrogen bonding. ( b ). Pressure evolution of the measured positions of signals in the wavenumber range from 1,800–4,000 cm −1 . Symbols represent experimental data while lines represent calculated data from ref. 19 . Line thickness corresponds to signal intensity. Solid dark blue symbols correspond to experimental data reported in ref. 24 while solid light blue outlined symbols represent data measured in this work. Blue and magenta highlighted fields correspond to measured strong absorption associated with the molecular and the ionic phase respectively. ( c ) Comparison of theoretically calculated IR absorption spectra and their evolution with pressure. ( d ) Comparison of IR absorption spectra measured at 67 GPa and calculated at 60 GPa. Full size image We note that the measured spectrum of the known molecular phase, P2 1 2 1 2 1 , as well as its pressure evolution, remained in good agreement with the previously reported experimental [24] and theoretical data [19] for both low- and high-frequency spectral regions ( Fig. 2b,d and Supplementary Fig. 1A ). Such high degree of consistency between experimental and simulated spectra validates theoretical models implemented in our study as well as in ref. 19 . Raman scattering Disappearance of strong NH 3 -derived vibrons with simultaneous appearance of two new strong signals in Raman spectra: a broadband at ~3,100 cm −1 and well-defined peak at ~3,695 cm −1 indicating major changes of ‘N–H’ stretching modes of ammonia. We also observed significant changes in the spectral range corresponding to ‘N–H’ bending modes (~1,600–2,100 cm −1 ). In particular, characteristic modes of NH 3 species (~1,600 cm −1 ) disappeared while new signals appeared around ~1,800–2,100 cm −1 ( Fig. 3a ). The measured Raman scattering spectra are consistent with the available experimental data [25] in the spectral region of internal ‘N–H’ stretching vibrations (>3,000 cm −1 ). To our best knowledge, no experimental report on low-frequency modes (<3,000 cm −1 ) has been previously reported in the pressure range of this study. We thus compared the measured frequencies with those calculated for the ionic Pma2 phase ( Fig. 3b,c and Supplementary Fig. 1C ). On that basis, we associated the new broad signal (~3,100 cm −1 ) with ‘N–H’ stretching while the new signals at lower frequency (~1,800 cm −1 ) with bending vibrons of both ammonium (NH 4 + ) and amide (NH 2 − ) species. 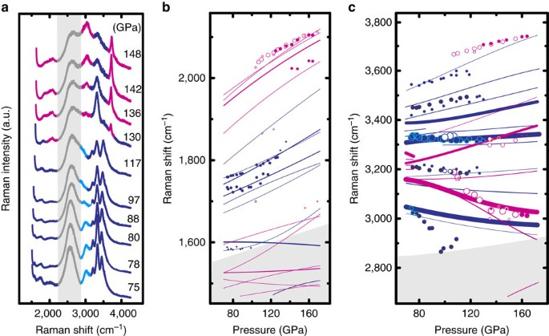Figure 3: Raman scattering study in solid ammonia under pressure. (a) Representative Raman spectra of solid ammonia collected at different pressures (fragment of high-frequency spectral range). The signal related to the second order Raman signal of diamond anvil is grey shadowed. Colours depict features attributed to molecular phase (blue (royal)) and ionic (magenta) phases, respectively. The light blue highlighted peak corresponds to the Raman signal associated with the most labile hydrogen bonding. (b,c) Pressure evolution of Raman shifts. Grey shadowed regions correspond to the signal of diamond anvil (the first and the second order Raman inbandc, respectively). Lines and symbols correspond to calculated and experimentally measured data. Thickness of lines and size of symbols correspond to intensities of presented data. The rest of colours and symbols designation is similar to that ina. Figure 3: Raman scattering study in solid ammonia under pressure. ( a ) Representative Raman spectra of solid ammonia collected at different pressures (fragment of high-frequency spectral range). The signal related to the second order Raman signal of diamond anvil is grey shadowed. Colours depict features attributed to molecular phase (blue (royal)) and ionic (magenta) phases, respectively. The light blue highlighted peak corresponds to the Raman signal associated with the most labile hydrogen bonding. ( b , c ) Pressure evolution of Raman shifts. Grey shadowed regions correspond to the signal of diamond anvil (the first and the second order Raman in b and c , respectively). Lines and symbols correspond to calculated and experimentally measured data. Thickness of lines and size of symbols correspond to intensities of presented data. The rest of colours and symbols designation is similar to that in a . Full size image In contrast to measured spectra, our calculated spectra yielded no Raman active mode around~3,695 cm −1 for Pma2 phase. However, during pressure release run of the same sample, we found that the measured signal was significantly less intensive in comparison with other signals belonging to Pma2 phase ( Supplementary Figs 3,4 and Supplementary Discussion ). At the moment, we have no unambiguous explanation for the origin of the observed signal except the one having relation to specific experimental conditions like inhomogeneity of pressure. There are certain unavoidable limitations of theory in simulating experimental conditions. Theory deals with an ideal crystal structure while pressure gradients (deviatoric stresses), kinetics effects (slow diffusion) and accumulation of defects and so on, may drive distortion of crystal structure, especially during phase transformation, and hence activate some modes (by breaking certain selection rules). This may also apply to fundamental molecular modes. This explains why not all signals can be absolutely well reproduced by theoretical calculations. Comparison of the measured X-ray diffraction and spectroscopic data with theoretically calculated results yields a good agreement providing strong evidence for the pressure-induced molecular to ionic phase transition in ammonia. We thus report ammonia as a first experimentally confirmed example of pressure-induced complete ionic disproportionation of a binary HB compound. Indeed, it stands out from other HB solids in which ionic disproportionation is predicted to exhibit a dynamical (for example, H 2 O (ref. 26 ), H 2 S (ref. 27 )) or still an incomplete character under extreme conditions (for example, H 2 O (ref. 18 )). We now focus on a possible mechanism of the disproportionation process in ammonia. Structural comparison of the low-pressure molecular and the high-pressure ionic phases reveals crucial clues on the underlying mechanism of the observed phase transition. First, from the structural point of view ( Supplementary Fig. 5 ), the transition from the molecular to the ionic phases involves a shift of closed packed planes: it thus resembles the well-known reversible hcp-to-fcc phase transition observed in relatively simple (for example, noble gases [28] ) and more complex systems (yttrium and other lanthanide trihydrides [29] , [30] ). Indeed, the experimentally observed continuous character of the intensity change of the hkl(020) (molecular) and the hkl(210) (ionic) reflections ( Fig. 1a ) provides direct evidence on the engagement of those close packed layers and it also corroborates a quasi hcp-to-fcc nature of the transition. Second, in the molecular phase (P2 1 2 1 2 1 ), one can distinguish two types of hydrogen bonding with respect to the angle in the ‘N–H N’ fragment: an ‘intra-plane’ bond with the angle value of ~158° and an ‘inter-plane’ bond with the angle value close to ~169° ( Supplementary Fig. 5 ). According to experimental spectroscopic data, the most labile hydrogen bond, the one exhibiting strong softening in both the IR and Raman spectra, is located between the closely packed layers. We therefore call this bond ‘inter-plane’. We found that a gradual, pressure-induced elongation of the covalent component (‘N–H’) leads to complete proton transfer from one neutral NH 3 molecule of to the other, resulting in formation of the NH 4 + /NH 2 − pairs at ~127 GPa. The resulting Pma2 arrangement, features a remarkably low anisotropy of the hydrogen bonds (~165° and ~163° for ‘inter-‘ and ‘intra’plane type, respectively), much lower than in the case of molecular P2 1 2 1 2 1 , phase. At this point, one can clearly distinguish two major stages governing the observed molecular to ionic phase transition: the first is the process of ‘interplane’ proton transfer; the second is the stage of structural rearrangement (in particular, sliding of the closely packed layers). Based on the spectroscopic observations, we believe that the proton transfer ‘starts’ first at pressures well below the observed actual structural transformation. Nonetheless, a definite answer to the question on which of the stages drives the phase transition is a matter of discussion, and, at this moment, falls beyond the scope of the present paper. We note, however, that the experimentally observed reversibility of the transformation points to the fact that ‘interplane’ proton transfer can effectively occurs within layers of quasi closely packed nitrogen atoms in either P2 1 2 1 2 1 or Pma2. Intuitively, a gradual ionization of the initial molecular P2 1 2 1 2 1 phase with subsequent structural transformation to Pma2 phase also looks plausible; however, at this moment, we are ruling this possibility out. If the assumed reaction path was realized via an intermediate phase, ionized via proton transfer with the P2 1 2 1 2 1 symmetry preveserved, one would have expected signs of disproportionation/ionization at pressure range well preceding the pressure of the structural phase transition observed in the XRD data (the appearance of NH 4 + - and NH 2 − -related gives highly specific IR absorption bands and Raman signals, which is difficult to omit). Instead, both the spectroscopic and the structural changes were observed in a narrow pressure range of 5–10 GPa indicating a simultaneous character of the transformation. Furthermore, according to our DFT calculations, such intermediate ionic phase (ionic P2 1 2 1 2 1 ) is dynamically unstable below 50 GPa and relaxes spontaneously to the known phase (molecular P2 1 2 1 2 1 ). On the contrary, an intermediate molecular phase of Pma2 symmetry is meta-stable below 50 GPa featuring a local minimum in total energy profile: moreover, our calculation indicates that such meta-stable phase is separated from the ionic Pma2 phase by an exceedingly small, yet distinct, energy barrier. For better understanding the proposed phase transition, we introduce a hypothetical molecular phase with the effective symmetry Pc, which is derived directly from the Pma2 ( Fig. 4 ). This model structure exhibits a number of advantageous features allowing for qualitative and quantitative analysis of the molecular to ionic phase transition. It shares features of both the ionic phase (arrangement of the nitrogen atoms, the shape and volume of the unit cell are effectively identical as in the ionic phase) and the molecular one (easily distinguishable, isolated ammonia molecules). We note, that the difference between the hypothetical molecular (Pc) and the experimental molecular (P2 1 2 1 2 1 ) arises only from different NH 3 packing–quasi fcc versus quasi hcp, respectively. Calculated enthalpy corroborates the intermediate character of the Pc phase ( Fig. 4 ). Furthermore, at this point, one can easily distinguish two types of energy contribution. Since we assume the similarity (with respect to crystal structure) of the Pma2 and Pc phases, the enthalpy difference (ΔH*) reflects the energy required for the proton transfer. The remaining difference in energy (between the model molecular phase (Pc) and experimentally observed one (P2 1 2 1 2 1 ) is associated with the process of structural rearrangement. 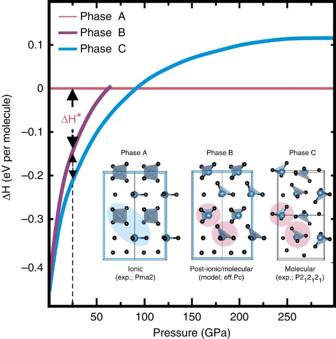Figure 4: Description of hypothetical intermediate phase. Calculated curves for enthalpy difference (ΔH) for the three considered phases of ammonia. Enthalpy of the high-pressure, ionic Pma2 (Phase A) establishes the reference (zero) line. Note the convergence of the absolute enthalpy of the experimental molecular P212121(Phase C) with the enthalpy of the hypothetical model molecular Pc (Phase B) with the decreasing pressure. As an example, the enthalpy difference (ΔH*) corresponding to the proton transfer contribution calculated at pressure of 25 GPa is shown. Insets illustrate schematically the structural similarities of the three phases considered. Figure 4: Description of hypothetical intermediate phase. Calculated curves for enthalpy difference (ΔH) for the three considered phases of ammonia. Enthalpy of the high-pressure, ionic Pma2 (Phase A) establishes the reference (zero) line. Note the convergence of the absolute enthalpy of the experimental molecular P2 1 2 1 2 1 (Phase C) with the enthalpy of the hypothetical model molecular Pc (Phase B) with the decreasing pressure. As an example, the enthalpy difference (ΔH*) corresponding to the proton transfer contribution calculated at pressure of 25 GPa is shown. Insets illustrate schematically the structural similarities of the three phases considered. Full size image We therefore consider the Pc phase as a good approximation to the experimental molecular phase and use it to model NH 3 /NH 3 to NH 4 + /NH 2 − transition mechanism and calculate the associated energy changes. Because of the intermediate character of the hypothetical Pc phase (both energetically and structurally), a simple proton transfer from one NH 3 molecule to a neighbouring one results in a smooth transition from molecular to ionic phase ( Fig. 5a ). To investigate the abovementioned implications of pressure-induced H + transfer, resulting in NH 3 /NH 3 to NH 4 + /NH 2 − transition, we have modelled the process between the NH 3 molecules in molecular phase and in 1-, 2- and 3-dimensional solids ( Supplementary Figs 6–9 and Supplementary Discussion ). The resulting energy profiles for 3-dimensional solid are given in Fig. 5b . 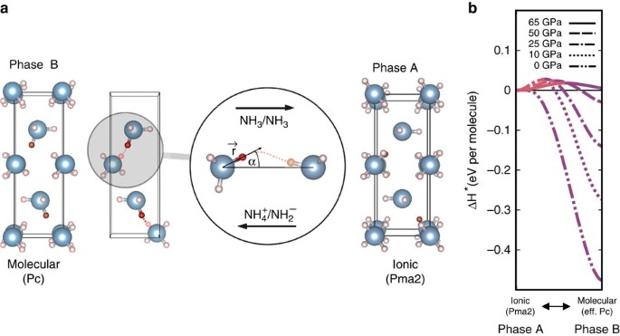Figure 5: Modelling the mechanism of the autoionization in solid ammonia. (a) Schematic illustration of the computational scheme used to determine the minimal energy path of H+transferred during the molecular to ionic phase transition. Red spheres indicate the ‘bridging’ hydrogen atoms transferred from one NH3molecule to the other resulting in formation of the NH4+/NH2−ionic pair. (b) Calculated energy profiles depicting the enthalpy changes, ΔH*, associated with the proton transfer between experimentally observed ionic phase and the proposed molecular phase of ammonia. Here, the calculated enthalpy of the ionic phase is set to 0. At the low-pressure limit (P→0 GPa) the ionic phase (Pma2) is calculated to be dynamically unstable. Upon relaxation, it spontaneously transforms into phase exhibiting purely molecular character. However, upon compression, the ionic phase stabilizes and already at P ~10 GPa, our model predicts formation of two minima, separated by an energy barrier. At lower pressures, the molecular minimum is strongly favored. According to the proposed model, transition from Phase A to Phase B occurs spontaneously at the low-pressure limit. With increasing pressure, the model molecular Phase B destabilizes. At ~62 GPa, the two structures exhibit enthalpy degeneracy and at P>70 GPa spontaneously transforms into the ionic one. Both structures remain separated by a small, yet persistent energy barrier of ~10 meV (calculated per NH3molecule). Figure 5: Modelling the mechanism of the autoionization in solid ammonia. ( a ) Schematic illustration of the computational scheme used to determine the minimal energy path of H + transferred during the molecular to ionic phase transition. Red spheres indicate the ‘bridging’ hydrogen atoms transferred from one NH 3 molecule to the other resulting in formation of the NH 4 + /NH 2 − ionic pair. ( b ) Calculated energy profiles depicting the enthalpy changes, ΔH*, associated with the proton transfer between experimentally observed ionic phase and the proposed molecular phase of ammonia. Here, the calculated enthalpy of the ionic phase is set to 0. At the low-pressure limit (P→0 GPa) the ionic phase (Pma2) is calculated to be dynamically unstable. Upon relaxation, it spontaneously transforms into phase exhibiting purely molecular character. However, upon compression, the ionic phase stabilizes and already at P ~10 GPa, our model predicts formation of two minima, separated by an energy barrier. At lower pressures, the molecular minimum is strongly favored. According to the proposed model, transition from Phase A to Phase B occurs spontaneously at the low-pressure limit. With increasing pressure, the model molecular Phase B destabilizes. At ~62 GPa, the two structures exhibit enthalpy degeneracy and at P>70 GPa spontaneously transforms into the ionic one. Both structures remain separated by a small, yet persistent energy barrier of ~10 meV (calculated per NH 3 molecule). Full size image Although height of the energy barrier remains relatively small for all pressures, its presence effectively precludes N–H N bond symmetrization, in contrast to highly compressed water, for which the symmetrization occurs at P~100 GPa (ref. 31 ). Note also the increasing contribution of the structural rearrangement process. In contrast to lower pressures at which the major part of energy is consumed for hydrogen transfer, the crystal structure rearrangement seems to become determinative at higher pressures. This assumption qualitatively account for the experimentally observed coexistence of two phases. According to our XRD and Raman spectroscopy studies, the molecular phase persists up to at least 172 GPa ( Fig.1e inset). Moreover, in an additional XRD runs, a significant amount of P2 1 2 1 2 1 phase was still detected, even up to the highest pressure of ~203 GPa ( Supplementary Fig. 10 and Supplementary Discussion ). Finally, we note that the P2 1 2 1 2 1 →Pma2 transition is predicted to occur at a pressure close to 90 GPa (ref. 19 and this study Fig. 4 ) yet is experimentally observed at pressures close to 130 GPa. This discrepancy may in part be due to athermal nature of the calculations where all entropic contributions are neglected. In conclusion, ammonia presents a qualitatively new picture of HB solid under pressure. Our detailed study provides first experimental evidence of the pressure-induced complete proton transfer resulting in the formation of the ionic phase (formation of NH 4 + /NH 2 − pairs) in compressed solid ammonia. The proton transfer is found to be a continuous and reversible process starting already at ambient pressure and completing at ~125 GPa. In fact, such a wide range of hydrostatic pressure required for proton transfer is unprecedented. The final stage of autoionization process is found to be accompanied by the quasi first order transformation resembling a quasi hexagonal to cubic structural phase transition. Our theoretical calculations provide a deep insight into the mechanism underlying the observed phenomenon indicating no hydrogen-bond symmetrization on the whole reaction path and remarkably small energy barrier between competitive phases. An increasing energy cost of the structural rearrangement component to the total energy is suggested to account for the overall slowing down of the autoionization process confirmed by the experimental observation of the molecular form up to 203 GPa. This unique scenario has no analogy among other known simple HB system such as water (H 2 O), hydrogen halides (HCl, HBr and so on) or H 2 S for which compression leads to either hydrogen bonds symmetrization or decomposition. We hope that the reported experimental evidence on the new form of ammonia and the observed peculiar behaviour of hydrogen bonds under pressure will stimulate further experimental as well as further theoretical research on new forms of simple HB systems in general and in particular, on the conductive properties of the ionic ammonia, which may turn to be critical for better understanding the observed properties of giant planets in our solar system. Experimental methods Number of successful (pressure achieved>150 GPa) experiments:Raman—5 (including two pressure release runs). Re gaskets were used in two measurements, W gaskets were used in other three experiments. Combined (IR+Raman)—5 (all were carried out using W gaskets with Au-lining), XRD (synchrotron) measurements—6 (gasket materials: Re without Au-lining (2 measurements), W without Au-lining (four measurements)). Size of sample varied depending on the technique used. Generally for the XRD and Raman measurements samples were of ~10–12 μm initial thickness and~35 μm in diameter. For IR measurements, samples were significantly thinner (initial thickness ≲ 1 μm) in order to get better resolved spectrum, especially, in the region of strong absorption of N–H molecular vibrations. The Raman spectrum of diamond anvil was used for pressure calibration. Moreover, during XRD measurements ‘diamond-Raman-edge’ scale was cross-checked by pressure estimation from equation of state of gasket materials (W, Re or Au). Neither diamond anvils nor gaskets were subjected to any passivation. For experiments, samples of liquefied ammonia were loaded into diamond anvil cells in the temperature range 195–240 K. Beveled diamonds with a culet diameter of 100 μm (and less) were used to reach pressures above 1 mbar. Gasket holes were prepared using IR laser drilling. Angle dispersive X-ray diffraction studies were conducted at the Advanced Photon Source (HPCAT, GSECARS), Argonne National Laboratory, USA and European Synchrotron Radiation Facility (ID 9, ID 27). Raman scattering was excited using a 25 mW HeNe (632.8 nm) laser. Raman spectra were collected in backscattered geometry using a single imaging spectrometer HR460 (focal length 460 mm) equipped with a 900 grooves per mm grating, giving a resolution of ~1 cm −1 , notch filters (Keiser Optical Systems) and liquid nitrogen cooled CCD detection. IR absorption spectra were measured in transmission mode using Fourier transform IR) spectrometer (Bruker Equinox 55) equipped with a glow-bar source, KBr beamsplitter and MCT detector (HgCdTe). To avoid spectra contamination by strong absorption lines of H 2 O and CO 2 molecules from the air, sample chamber of the spectrometer was purged with dry nitrogen. Details of theoretical calculations All of the reported calculations were performed using density-functional-theory (DFT) with the Perdew-Burke-Ernzerhof parameterizations of the generalized gradient approximation, as implemented in the VASP (ver. 4.6), CASTEP and ABINIT codes. The 1s and 2s/2p electrons were included in the valence space for H and N atoms, respectively. For the plane-wave basis-set expansion, an energy cutoff of 750 eV was used. To sample the first Brillouin zone (FBZ), we used sufficiently dense Γ-centred k-point grids to achieve accurate sampling convergence. All structures were fully optimized until the forces acting on atoms converged to 0.001 eV/Å or less. We neglect ZPE contributions during the simulations. Lattice parameters and atomic positions were optimized by seeking a total minimum energy for the NH 3 unit cells based on density-functional theory and the plane-wave pseudopotential method. In order to perform the geometry optimization, the following thresholds were applied for a convergence window of two successive self-consistent steps: total energy change smaller than 1 × 10−6 eV/atom, maximum force per atom below 0.005 eV/Å, pressure smaller than 0.005 GPa, and maximum atomic displacement not exceeding 1 × 10−3 Å. The BFGS minimizer was employed to carry out the unit cell optimization. The quality of this basis set was kept fixed as the unit cell volume varied during geometry optimization. After obtaining the unit cell and atomic positions, the normal-mode vibrational analysis of NH 3 (P2 1 2 1 2 1 and Pma2) was performed with ab initio lattice dynamics. Calculations were performed using the PBE exchange-correlation functional. Brillouin-zone integration was performed according to the Monkhorst-Pack scheme with a dense mesh of k points, which gave convergence of all modes to a precision of better than 3 cm −1 . Pseudopotential errors in the frequencies were estimated at no more than 2% from a comparison of competitive pseudopotentials. The normal modes of the crystalline phases were determined from dynamical matrices calculated using density-functional perturbation theory). Raman and IR intensities were calculated using the formalism presented in refs 32 , 33 . How to cite this article : Palasyuk, T. et al. Ammonia as a case study for the spontaneous ionization of a simple hydrogen-bonded compound. Nat. Commun. 5:3460 doi: 10.1038/ncomms4460 (2014).